First evidence of a 200-day non-stop flight in a bird Being airborne is considered to be energetically more costly as compared with being on the ground or in water. Birds migrating or foraging while airborne are thought to spend some time resting on the ground or water to recover from these energetically demanding activities. However, for several decades ornithologists have claimed that some swifts may stay airborne for almost their whole lifetime. Here we present the first unequivocal evidence that an individual bird of the Alpine swift ( Tachymarptis melba ) can stay airborne for migration, foraging and roosting over a period of more than 6 months. To date, such long-lasting locomotive activities had been reported only for animals living in the sea. Even for an aerodynamically optimized bird, like the Alpine swift, flying requires a considerable amount of energy for continuous locomotive control. Our data imply that all vital physiological processes, including sleep, can be perpetuated during flight. Animals exploring the open airspace are confronted with somehow similar requirements as animals living in the sea [1] . But, remaining in or on the water does not implicitly need any energy expenditure, because weight can be balanced passively by the buoyancy of the body. In contrast, the low density of the air requires that a constant flow across the wings must be maintained to produce lift to stay airborne. For vertebrates, being airborne is considered to be energetically more costly compared with being on the ground or in water [2] . Therefore, birds migrating or foraging on the wing are expected to spend some time resting on the ground or on water to recover from these energetically demanding activities [3] . Flying was considered as a behaviour that does not go along with sleep or rest, because there is a constant need for an active control of flight to account for varying conditions of the air flow around the wings [4] . It is well known that sea birds can soar for several days while foraging. However, from time-to-time they dive or stay on water to feed or rest [5] , [6] . Since several decades ornithologists have claimed that some swifts may stay on the wing for almost their whole lifetime except for breeding [7] , [8] . This claim was based solely on radar tracks from aerial roosting flights at night of common swifts ( Apus apus ) during their breeding period [9] , [10] . Based on these observations, it has been assumed that these birds might stay on their wing all their life, except when breeding and feeding their chicks [11] . Our study species, the Alpine swift ( Tachymarptis melba ), is one of the largest swift species. Like all swifts, it feeds on aerial plankton. Their morphology and flap-gliding flight style is adapted to maximise flight efficiency [12] . Alpine swifts breeding in Switzerland are trans-Sahara migrants, assumed to spend the winter in Western Africa [13] . Neuroscientists investigating the problem of sleep did not find evidence for a full recovery sleep in flight [14] . It was pointed out that periods of undisturbed post-flight recovery sleep may be essential for maintaining adaptive brain function during wakefulness [15] . Although it had been claimed for several decades that swifts, and specifically common swifts, stay on the wing for the most part of their life, no data are available at the individual level confirming such long-lasting flights so far. We here investigate the year-round temporal and spatial movement patterns of the Alpine swift. Their activity pattern reveals that they can stay airborne continuously throughout their non-breeding period in Africa and must be able to recover while airborne. To date, such long-lasting locomotive activities had been reported only for animals living in the sea [16] , [17] . Spatial and temporal pattern Six Alpine swifts were equipped at a breeding site in Switzerland with tags logging light for information on their whereabouts [18] and acceleration for measuring their activity [19] . After their return to the breeding site in the following year, three of the six birds were recaptured. Based on the stored data, we could reconstruct their non-breeding movements ( Fig. 1 ) and activity pattern ( Figs 2 and 3 ) over a period of at least 7 months. Because nest sites are inside a building (in the dark), nest visits of the birds during daytime were easily detectable by the abrupt change in the light level. When the birds are exposed to natural light conditions, light levels change gradually during twilight. The light-based geolocation confirms the supposed winter quarters in West Africa ( Fig. 1 ). In spring, after having crossed the Sahara they spend some time in Northern Africa and Southern Spain. 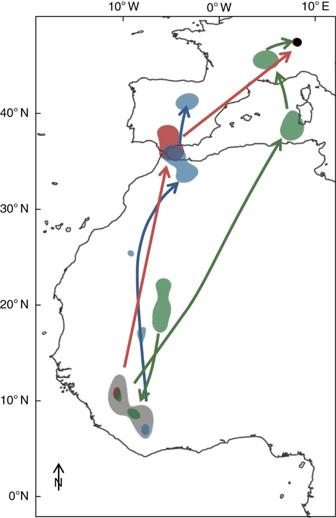Figure 1: Migration routes and non-breeding range of three Alpine swifts breeding in Switzerland. The map shows South-Western Europe and Western Africa. Each colour represents an individual (blue=I1, green=I2, red=I3). The black point indicates the breeding site, coloured areas in Africa mark the centre (75%-kernel) of the individual wintering ranges and the grey area represents the 50%-kernel of all three birds together. 50% kernel densities are given for stopover sites along the migration route. Arrows indicate spring migration routes and only the last step of the autumn migration of one individual, because movements occurred mainly during equinox, when no latitudinal information could be derived. Map and kernel projection refers to WGS_1984 UTM_Zone 31N. Figure 1: Migration routes and non-breeding range of three Alpine swifts breeding in Switzerland. The map shows South-Western Europe and Western Africa. Each colour represents an individual (blue=I1, green=I2, red=I3). The black point indicates the breeding site, coloured areas in Africa mark the centre (75%-kernel) of the individual wintering ranges and the grey area represents the 50%-kernel of all three birds together. 50% kernel densities are given for stopover sites along the migration route. Arrows indicate spring migration routes and only the last step of the autumn migration of one individual, because movements occurred mainly during equinox, when no latitudinal information could be derived. Map and kernel projection refers to WGS_1984 UTM_Zone 31N. 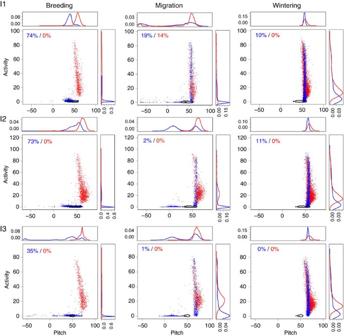Figure 2: Distribution of individual half-hour mean values for pitch and activity. Data are divided into three time periods (breeding, migration and wintering). Dates of the time periods are given inFig. 3. Migration includes stopover periods. Red colour represents data recorded during daytime and blue during darkness (night or inside a building or cave). Given are scatterplots (pitch vs activity) and density distributions of pitch (above) and activity (right) for each period and individual (I1, I2 and I3). The polygon (black line) in the scatterplot represents the 5%-kernel (95% of the range) density area of the individually defined reference area for resting. Percentages given in the upper left corner indicate the number of points inside the reference area for dark (blue) and light (red) phases. Full size image Figure 2: Distribution of individual half-hour mean values for pitch and activity. Data are divided into three time periods (breeding, migration and wintering). Dates of the time periods are given in Fig. 3 . Migration includes stopover periods. Red colour represents data recorded during daytime and blue during darkness (night or inside a building or cave). Given are scatterplots (pitch vs activity) and density distributions of pitch (above) and activity (right) for each period and individual (I1, I2 and I3). The polygon (black line) in the scatterplot represents the 5%-kernel (95% of the range) density area of the individually defined reference area for resting. Percentages given in the upper left corner indicate the number of points inside the reference area for dark (blue) and light (red) phases. 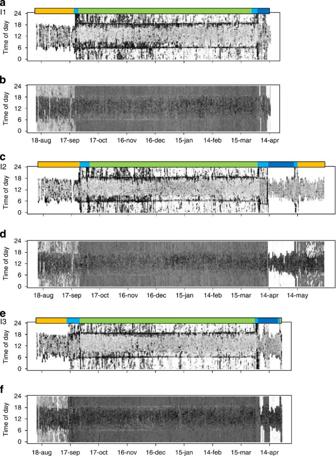Figure 3: Time series of the relative activity pattern and pitch axis for three individual Alpine swifts. For each individual (I1, I2 and I3) half-hour means for activity (a,c,e) and pitch (b,d,f) are shown. Increasing shading indicates increasing activity and pitch values closer to a horizontal position, respectively. The coloured bars above the activity patterns indicate the different time periods: yellow=breeding, light blue=active migration, dark blue=stopover site and green=sub-Saharan wintering site. Full size image Figure 3: Time series of the relative activity pattern and pitch axis for three individual Alpine swifts. For each individual (I1, I2 and I3) half-hour means for activity ( a , c , e ) and pitch ( b , d , f ) are shown. Increasing shading indicates increasing activity and pitch values closer to a horizontal position, respectively. The coloured bars above the activity patterns indicate the different time periods: yellow=breeding, light blue=active migration, dark blue=stopover site and green=sub-Saharan wintering site. Full size image Activity pattern We compared acceleration data between the breeding, the migration and the wintering periods and dark and light phases as recorded by the light sensor ( Fig. 2 ). All three individuals provided very similar patterns, but some differences in absolute values. During the breeding period, Alpine swifts are known to spend the nights roosting in the colony often close to their nest [17] . The clearly twofold distribution of pitch and activity ( Fig. 2 ) confirms these observations. Flight is characterized by a high variability in activity and a narrow range in pitch, and resting by low activity and a large variance in pitch. The migration period includes both flapping activity during the day and night as well as resting with very low pitch values. During the wintering period flapping activity is generally lower during the night than during the day, but consistently and significantly higher than that during the night at the breeding site. Low pitch values typical for resting is not represented at all ( Fig. 2 ). To quantify the potential amount of resting within each time period, we estimated the overlap of 30 min mean pitch and activity values with an individual reference kernel for resting. Because resting positions can be similar to flight positions while soaring or gliding, there is an overlap between aerial roosting and resting positions in two of the three individuals ( Fig. 2 ). The overlap between the resting reference kernel and the values during the wintering period varies between 0–11%. Nevertheless, the temporal activity pattern in combination with the pitch values do not give evidence for resting events during the wintering period. In all three individuals, the patterns of both parameters consistently differ before and after the crossing of the Sahara desert. In contrast to the breeding and some stopover periods, there is always activity at night during the wintering period ( Fig. 3a,c,e ). Pitch values during the wintering period show little variability and are very consistent over the whole range of activity ( Fig. 3b,d,f ; cf. Fig. 2 ). Low pitch values reveal that the birds resting during the stopover period in the Mediterranean area are most probably hanging on cliffs or trees. Twilight activity There is a distinct pattern in diurnal activity during the sub-Saharan wintering period ( Fig. 3a,c,e ). All three individuals show a pronounced and well-synchronised increase in flapping activity around dawn and dusk ( Fig. 4 ). In the morning, the flapping activity boosts quickly and peaks around civil twilight and then fades out into the day. In the evening, the flapping activity gradually increases towards sunset and decreases rapidly around civil twilight. This diurnal activity pattern can be observed during most, but not all twilight events ( Fig. 3a,c,e ). 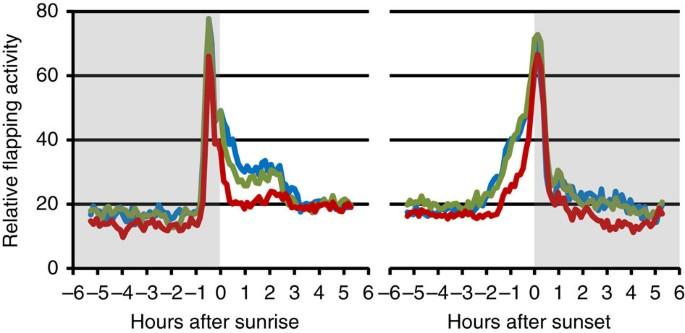Figure 4: Mean course of the relative flapping activity in relation to hours before and after sunset and sunrise. Only data from the time in the sub-Saharan wintering site were included. Sunrise and sunset refers to a sun-elevation angle of −2.2°. Each colour represents an individual (blue=I1, green=I2 and red=I3). Figure 4: Mean course of the relative flapping activity in relation to hours before and after sunset and sunrise. Only data from the time in the sub-Saharan wintering site were included. Sunrise and sunset refers to a sun-elevation angle of −2.2°. Each colour represents an individual (blue=I1, green=I2 and red=I3). Full size image To our big surprise, the Alpine swifts change their flight behaviour drastically between the breeding period, active migration and the non-breeding stage in Africa. The activity pattern in combination with the pitch values allows distinguishing between periods of flying and resting ( Fig. 2 ). During daytime, all individuals showed an activity and pitch pattern, which excludes resting on the ground. At night, the low flapping activity during the wintering period is in accordance with nocturnal radar recordings of common swifts performing elongated gliding flights without wing flapping during their roosting flights [9] , [10] . Thus, nocturnal roosting on the wing is characterized by long gliding intervals (with almost zero activity) and stable pitch position. This combination can be observed mainly during the wintering period and to some extent during migration, but rarely during breeding ( Fig. 2 , blue points). In two birds there is some overlap between the reference kernels for resting with the nocturnal data during the wintering period. If this overlap would indicate resting on the ground during wintering, we would have to assume that these birds were always resting in exactly the same pitch position as during flight, because other pitch values are lacking ( Fig. 2 ). As this is very unlikely, we conclude that all three individuals were most probably constantly on their wings during their stay in the sub-Saharan African winter quarters. We cannot rule out that Alpine swifts may interrupt their flight for a few minutes. Nevertheless, they must be able to accomplish all vital physiological functions in flight over a period of several months. Roosting common swifts hanging on trees have been observed in Europe, in relation to cold weather [20] . This gives a hint, that aerial roosting is driven by food availability, which might restrict aerial roosting of the large Alpine swifts to the equatorial region. A dawn and dusk ascent described recently for common swifts [21] let us assume that the observed increase in activity at dawn and dusk implies a corresponding ascent in the Alpine swifts. The function of such an ascent is not clear yet. Based on the radar data, which also recorded insect densities, it could be ruled out that the ascent was related to foraging [21] . Birds are homoeotherms with the highest basal metabolic rate and with the highest metabolic rates attained during endurance exercise among vertebrates [22] . To date, long-lasting flights have been investigated under the aspect of fasting during flight [22] . Recent studies showed that immune responses seem to be affected by long-lasting flights [23] . Alpine swifts feed on the wing and might be able to compensate such negative effects on immune defence. In addition, such long-lasting flights raise the question of how or whether these birds sleep. For many decades sleep has been considered as an unavoidable necessity to restore at least some of the physiological functions of the brain [24] . In Alpine swifts there seems to be no necessity for physical inactivity to maintain any of the relevant physiological processes. However, our data indicate that there are distinct periods of increased and decreased activity, which could go along with some kind of sleep in flight. It has been argued that locomotive control of flight is possible in slow-wave sleep, either unihemispherically as observed in dolphins or even bihemispherically [14] . Various birds carrying out long-distance flights are able to reduce sleep without the need for compensatory sleep afterwards. However, they still do sleep for some time and some other birds do show some kind of sleep deprivation after long-distance flights [14] , [15] , [22] . Although the sample size contains only three individuals, the consistent results confirm clearly that swifts do at least to some extent sleep while airborne and demonstrate that sleep deprivation does not necessarily have to occur after long-lasting flights. As a consequence, the whole organism must be maintained in flight, which has important implications for further models of sleep and other aspects of recovery, as well as for locomotive control of flight and the cost of flight in general. From the evolutionary aspect, we are interested to uncover the causes for this extraordinary behaviour. Study design Six Alpine swifts were caught in a breeding colony in Baden (Switzerland, 47°28.3′ N, 8°18.6′E) and equipped with data loggers. Birds in this colony are regularly captured and recaptured for ringing. Ringing and logging permission was issued by the Swiss Federal Office for the Environment in accordance with the national guidelines (FVO RT 4.03). We defined the breeding period as the time interval between arrival and departure from the breeding site. We used a new kind of data logger weighing 1.5 g, including harness (1.5% of the body weight), programmed to record intensity of blue light and static and dynamic acceleration data every 4 min. A single acceleration sample consisted of 32 consecutive measurements of the acceleration along the z axis of the sensor with a sampling frequency of 10 Hz. Due to the limited memory capacity, only the mean of a sample and the sum of the absolute differences between consecutive data points over the whole sample (named as ‘activity’) were stored, together with a single value for blue light. The mean value represents the static acceleration and therefore provides a relative measure of the deflection of the bird’s dorsoventral axis relative to the gravitational vector. As the amount of roll movements around the longitudinal axis on either side tend to level out while flying, the mean of the acceleration data reflects the inclination of the longitudinal axis (named as ‘pitch’). Data analysis For the calibration of the acceleration sensor, we collected reference data for the mean pitch values in relation to the absolute angle of the pitch by a static experiment in the laboratory ( Fig. 5 ). In addition, we used a different firmware recording data continuously with a sampling frequency of 10 Hz. To collect data on free-flying birds, we mounted two of these loggers on breeding individuals. Due to limited storage capacity, data on free-flying birds were collected for 12 h only. The raw data represent wing beat patterns very similar to known patterns from radar measurements ( Fig. 6 ) [9] . From these data, we simulated mean pitch and activity values for time intervals of 3.2 s in accordance to the sampling intervals of the loggers used for the year-round monitoring ( Fig. 7 ). The raw data was then subdivided into three categories (‘gliding’, ‘flapping’ and ‘resting’) by a careful visual inspection of the data. By comparing the value ranges of pitch and activity for the three categories, it was possible to characterize the three categories by means of the acceleration data. Pitch values from the A/D-converter were not transformed to angular values, because the exact inclination angle of the longitudinal axis could not be measured after the sensor was mounted on the bird. Activity accumulates all movements accelerating the body up and down, and typically represents the amount of wing beats ( Fig. 6 ). The selected measurement interval and data compression was a compromise between the memory capacity, battery lifetime and the temporal resolution of the activity data. Three examples of raw time series data as recorded during the year-round monitoring are given in Fig. 8 . 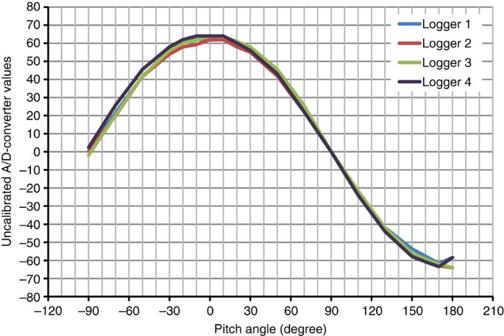Figure 5: Acceleration sensor validation. Static acceleration (pitch) from four test loggers (logger 1–4) was recorded in relation to the absolute pitch angle. Measurements were taken in the laboratory in the local gravitational field in steps of 10°. Each position was sampled over 2 min with a sampling frequency of 25 Hz. Figure 5: Acceleration sensor validation. Static acceleration (pitch) from four test loggers (logger 1–4) was recorded in relation to the absolute pitch angle. Measurements were taken in the laboratory in the local gravitational field in steps of 10°. Each position was sampled over 2 min with a sampling frequency of 25 Hz. 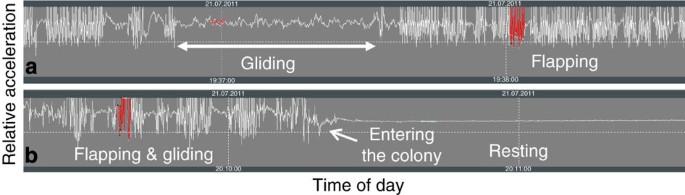Figure 6: Test data from a free-flying Alpine swift at the breeding colony in Switzerland. Given are continuous acceleration data (cf.Fig. 5) recorded at 10 Hz. Both panels show data from about 2 min. The upper graph (a) shows free flight with phases of wing flapping and gliding. The lower graph (b) shows the moment where the bird enters the colony for resting during the night. Intervals marked with red represent sample intervals corresponding to the time interval collected every 4 min over the whole year. The mean and the sum of the absolute difference between consecutive points of such a sample (32 data points) were stored. Full size image Figure 6: Test data from a free-flying Alpine swift at the breeding colony in Switzerland. Given are continuous acceleration data ( cf. Fig. 5 ) recorded at 10 Hz. Both panels show data from about 2 min. The upper graph ( a ) shows free flight with phases of wing flapping and gliding. The lower graph ( b ) shows the moment where the bird enters the colony for resting during the night. Intervals marked with red represent sample intervals corresponding to the time interval collected every 4 min over the whole year. The mean and the sum of the absolute difference between consecutive points of such a sample (32 data points) were stored. 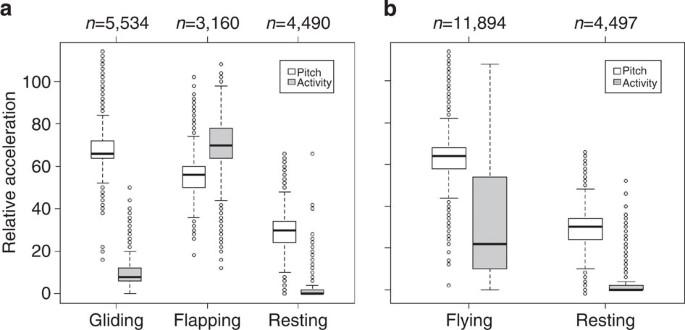Figure 7: Distribution of raw data. Pitch values and activity sampled from a single free-ranging Alpine swift in the breeding area equipped with a logger programed to collect data continuously (cf.Fig. 6). Pitch and activity was sampled in the same way as for the loggers used for the year-round monitoring (10 Hz for 3.2 s). Given are median, quartiles and outliers for selected periods corresponding to (a) gliding flight, flapping flight and resting, and (b) flying and resting. Inb, the samples during the flying period were collected randomly irrespective of gliding or flapping as it is the case for the data collected by loggers used for the year-round monitoring. ‘n’ represents the number of analysed measurement intervals of 3.2 s. Full size image Figure 7: Distribution of raw data. Pitch values and activity sampled from a single free-ranging Alpine swift in the breeding area equipped with a logger programed to collect data continuously ( cf. Fig. 6 ). Pitch and activity was sampled in the same way as for the loggers used for the year-round monitoring (10 Hz for 3.2 s). Given are median, quartiles and outliers for selected periods corresponding to ( a ) gliding flight, flapping flight and resting, and ( b ) flying and resting. In b , the samples during the flying period were collected randomly irrespective of gliding or flapping as it is the case for the data collected by loggers used for the year-round monitoring. 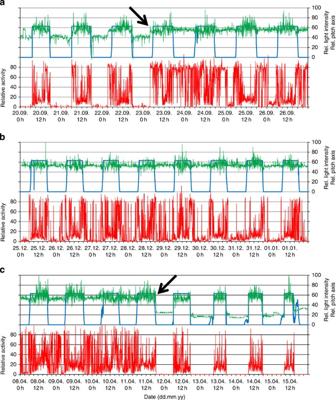Figure 8: Three examples of raw data as recorded during the year-round monitoring. Raw 4 min light (blue), activity (red) and pitch axis (green) data are presented for three selected periods from one individual. (a) The 7-day-period when the bird left the breeding site. The arrow marks the start of the migratory flight. The clear day–night activity pattern before the start of migratory flight is followed by an increased activity during night and day and a constant pitch axis typical for flight. (b) 7-day-period in the winter quarter with more or less variable activity and a constant pitch axis typical for flight. (c) The 7-day-period from the end of the Sahara crossing and arriving at a stopover site in the Mediterranean area (arrival indicated by arrow). The almost continuous activity is followed by a clear day–night rhythm of flight and rest. The pitch axis is much higher than before indicating an upward-directed position, most probably hanging on a cliff or tree. Scales given are uncalibrated A/D-converter values as derived directly from the logger. ‘n’ represents the number of analysed measurement intervals of 3.2 s. Full size image Figure 8: Three examples of raw data as recorded during the year-round monitoring. Raw 4 min light (blue), activity (red) and pitch axis (green) data are presented for three selected periods from one individual. ( a ) The 7-day-period when the bird left the breeding site. The arrow marks the start of the migratory flight. The clear day–night activity pattern before the start of migratory flight is followed by an increased activity during night and day and a constant pitch axis typical for flight. ( b ) 7-day-period in the winter quarter with more or less variable activity and a constant pitch axis typical for flight. ( c ) The 7-day-period from the end of the Sahara crossing and arriving at a stopover site in the Mediterranean area (arrival indicated by arrow). The almost continuous activity is followed by a clear day–night rhythm of flight and rest. The pitch axis is much higher than before indicating an upward-directed position, most probably hanging on a cliff or tree. Scales given are uncalibrated A/D-converter values as derived directly from the logger. Full size image For a comparison of the pitch and activity values between the different time periods, we calculated a reference kernel for the time when an individual rested on the ground based on the half-hour means ( cf. Figs 2 and 3 ). For this, only data recorded during the breeding period at night (2200–0400hours) were considered. For each time period, we calculated the percentage of data points within the reference resting kernel. Kernels were calculated with R version 2.15.0 (2012-03-30), package ‘adehabitatHR’, using the standard settings in the function ‘kernelUD’ with the options ‘h=LSCV’ and ‘kern=bivnorm’. For the analysis of the light data, we used the R-package ‘GeoLight’ [18] . The geographic positions for all three loggers was determined by using the median of the sun-elevation angle (−2.8°) derived from the Hill–Ekström calibration [18] . Stationary periods were calculated using the ‘cp’ function of the R-package ‘GeoLight’ with the options ‘quantiles=0.9’ and ‘days=10’. How to cite this article: Liechti, F. et al. First evidence of a 200-day non-stop flight in a bird. Nat. Commun. 4:2554 doi: 10.1038/ncomms3554 (2013).